Clozapine-induced agranulocytosis is associated with rareHLA-DQB1andHLA-Balleles Clozapine is a particularly effective antipsychotic medication but its use is curtailed by the risk of clozapine-induced agranulocytosis/granulocytopenia (CIAG), a severe adverse drug reaction occurring in up to 1% of treated individuals. Identifying genetic risk factors for CIAG could enable safer and more widespread use of clozapine. Here we perform the largest and most comprehensive genetic study of CIAG to date by interrogating 163 cases using genome-wide genotyping and whole-exome sequencing. We find that two loci in the major histocompatibility complex are independently associated with CIAG: a single amino acid in HLA-DQB1 (126Q) ( P =4.7 × 10 −14 , odds ratio (OR)=0.19, 95% confidence interval (CI)=0.12–0.29) and an amino acid change in the extracellular binding pocket of HLA-B (158T) ( P =6.4 × 10 −10 , OR=3.3, 95% CI=2.3–4.9). These associations dovetail with the roles of these genes in immunogenetic phenotypes and adverse drug responses for other medications, and provide insight into the pathophysiology of CIAG. Clozapine-induced agranulocytosis/granulocytopenia (CIAG) is a rare adverse drug event that occurs in 1% of treated individuals and can be fatal if not detected early [1] . As a result, clozapine is underused despite its superior efficacy and particular utility in treatment-resistant schizophrenia [2] . Our goal is to identify genetic risk factors for CIAG that could enable safer and increased use of clozapine. Because of the specific nature of this adverse drug response and the role of the major histocompatibility complex (MHC) in adverse drug responses, candidate gene studies have focused on human leukocyte antigen (HLA) alleles in CIAG [3] , [4] , [5] , [6] , [7] , [8] . A small exome sequencing study of CIAG was unrevealing [9] . While nominally significant HLA associations have been reported, no study to our knowledge has reported unequivocal statistical significance or the dissection of the complex linkage disequilibrium (LD) relationships in the MHC. 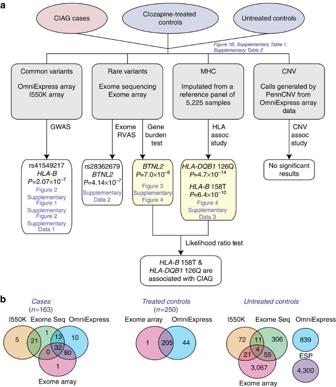Figure 1: Study design. Our study design consisted of looking for genetic associations with CIAG across the minor allele frequency spectrum. (a) First, we recruited CIAG cases (red circle) and both treated and untreated controls (blue circles). Next, we used multiple technologies to genotype variants including genotyping arrays for both common and rare variants, whole-exome sequencing, imputation of classical HLA four-digit alleles and amino acids in the major histocompatibility complex, and copy number variants. Finally, we performed association tests for each class of variants. Results that exceeded the multiple-testing threshold are coloured in yellow. References to figures and tables are listed in blue italics. (b) We used multiple technologies to genotype variants including whole-exome sequencing (green), exome array (pink), OmniExpress (blue) and Illumina 550K genome-wide arrays (orange). In addition, we used allele counts from the Exome Sequencing Project as extra control chromosomes (purple). As demonstrated by the Venn diagrams, the majority of cases (n=163) and treated controls (n=250) were genotyped on more than one platform. Using multiple ascertainment schemes, we assemble the largest CIAG cohort to date (163 cases, 54.0% never previously reported, Supplementary Table 1 ). We conduct a genome survey using whole-exome sequencing and genome-wide genotyping to test for association with CIAG ( Fig. 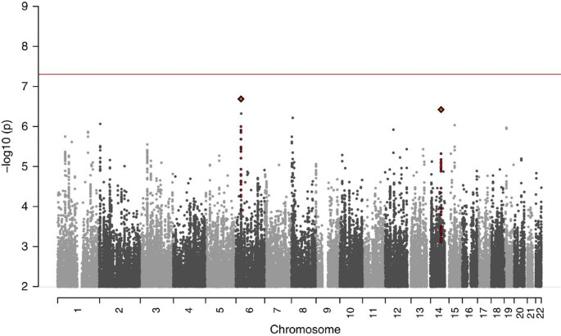Figure 2: GWAS Manhattan plot. We performed a genome-wide association study for 161 cases and 1,196 controls. We did not find any loci that exceeded the threshold for genome-wide significance of 5 × 10−8(red line). The most significant SNP is rs41549217, in an intron ofHLA-B(P=2.07 × 10−7, logistic regression). 1 , Supplementary Table 2 ). We show that CIAG is associated with two independent amino acid changes in HLA-B (158T) and HLA-DQB1 (126Q). However, the odds ratios (ORs) for these risk factors do not suggest immediate clinical application in predictive testing. Figure 1: Study design. Our study design consisted of looking for genetic associations with CIAG across the minor allele frequency spectrum. ( a ) First, we recruited CIAG cases (red circle) and both treated and untreated controls (blue circles). Next, we used multiple technologies to genotype variants including genotyping arrays for both common and rare variants, whole-exome sequencing, imputation of classical HLA four-digit alleles and amino acids in the major histocompatibility complex, and copy number variants. Finally, we performed association tests for each class of variants. Results that exceeded the multiple-testing threshold are coloured in yellow. References to figures and tables are listed in blue italics. ( b ) We used multiple technologies to genotype variants including whole-exome sequencing (green), exome array (pink), OmniExpress (blue) and Illumina 550K genome-wide arrays (orange). In addition, we used allele counts from the Exome Sequencing Project as extra control chromosomes (purple). As demonstrated by the Venn diagrams, the majority of cases ( n =163) and treated controls ( n =250) were genotyped on more than one platform. Full size image Genome-wide common variant association study We performed a genome-wide association study of 8,809,853 genotyped and imputed common variants in 161 CIAG cases (two additional cases had exome sequencing or exome array data) and 1,196 controls of European ancestry. After controlling for ancestry ( Supplementary Fig. 1 ), no loci exceeded genome-wide significance ( P <5 × 10 −8 , Fig. 2 ). Our sample size was powered to detect common genetic variants with effect sizes of clinical utility (for example, power was >99% for an OR>4 and MAF >10%; Supplementary Fig. 2 ). The single-nucleotide polymorphism (SNP) with the best evidence for association was in an intron in HLA-B (rs41549217, P =2.07 × 10 −7 , OR=4.66, 95% confidence interval (CI)=2.6–8.3, Supplementary Data 1 ). We specifically examined the distribution of P values of SNPs previously shown to be associated with immune-mediated diseases, but did not detect any enrichment ( Supplementary Fig. 3 ). Evaluation of copy number variation did not reveal any associations with CIAG. No protein encoded by a gene implicated by genome-wide association study (GWAS) is known to bind clozapine [10] . Figure 2: GWAS Manhattan plot. We performed a genome-wide association study for 161 cases and 1,196 controls. We did not find any loci that exceeded the threshold for genome-wide significance of 5 × 10 −8 (red line). The most significant SNP is rs41549217, in an intron of HLA-B ( P =2.07 × 10 −7 , logistic regression). Full size image Exome-wide rare variant association study We tested protein-coding variants (MAF <5%) for association using whole-exome sequencing data from 67 CIAG cases and 376 untreated population controls. For variants that were also genotyped on the exome array, we merged the sequencing data with exome array data from 81 CIAG cases and 3,294 controls of European ancestry. We also used raw count data from ~4,300 samples of European ancestry from the NHLBI Exome Sequencing Project as an additional control reference to increase statistical power [11] . The top finding is a low frequency missense variant in BTNL2 annotated as benign by PolyPhen-2 (rs28362679, P =4.14 × 10 −7 , OR=3.9, 95% CI=1.2–12.9, Supplementary Data 2 ). Next, we used a burden test to evaluate whether cases were more likely to be carriers of a functional variant in a gene compared with controls in the exome-sequencing data. We divided rare variants into different functional categories and MAF ranges and found that BTNL2 ( P =7.0 × 10 −8 ) was the only gene to exceed a conservative significance threshold of P =2.5 × 10 −6 , corresponding to a Bonferroni correction of 20,000 genes tested [12] ( Fig. 3 ). None of the protein products of these genes is known to bind clozapine [10] . The BTNL2 signal is driven by two independent variants: the top SNP noted above (rs28362679) and a conditionally independent missense variant annotated as benign by PolyPhen-2 (rs143211074; P =6.0 × 10 −6 , OR=4.4, 95% CI=1.10–17.8). These associations replicated using the exome array and NHLBI Exome Sequencing Project data ( Supplementary Fig. 4 ). BTNL2 is in the MHC region and is in strong LD with HLA-DQB1 and HLA-DRB1 , which have been associated with autoimmune diseases and adverse drug reactions including CIAG [7] , [13] . BTNL2 codes for the butyrophilin-like protein 2, a member of the immunoglobulin gene superfamily with a role in regulating T-cell activation [14] . Given its location in a region of very high LD, the BTNL2 association could implicate it directly or reflect indirect associations with classical HLA alleles. 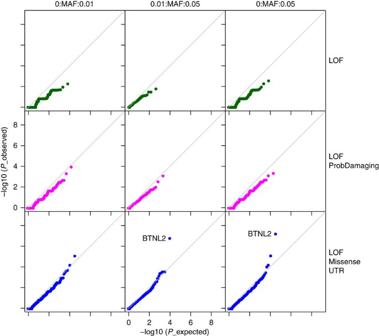Figure 3: Gene-burden test results. We evaluated whether cases were more likely to carry rare functional variants in a gene compared with controls using sequencing data from 67 cases and 376 controls. Variants were annotated using the variant effect predictor tool and divided into three sets of severity. The most severe category consists of loss-of-function (LOF) variants annotated as being nonsense and splice site (green). The intermediate category included all LOF variants as well as missense variants annotated as probably damaging by PolyPhen-2 (magenta). The least severe category consisted of all LOF, missense and untranslated region (UTR) variants (blue). We had varying minor allele frequency (MAF) cutoffs with the most restrictive being 0–1% MAF and the most inclusive being 0–5%. For each MAF and variant set, we assessed whether any genes deviated from expectation as demonstrated by the diagonal line. The only gene that showed enrichment wasBTNL2(P=7.0 × 10−8, Fisher’s exact test). Figure 3: Gene-burden test results. We evaluated whether cases were more likely to carry rare functional variants in a gene compared with controls using sequencing data from 67 cases and 376 controls. Variants were annotated using the variant effect predictor tool and divided into three sets of severity. The most severe category consists of loss-of-function (LOF) variants annotated as being nonsense and splice site (green). The intermediate category included all LOF variants as well as missense variants annotated as probably damaging by PolyPhen-2 (magenta). The least severe category consisted of all LOF, missense and untranslated region (UTR) variants (blue). We had varying minor allele frequency (MAF) cutoffs with the most restrictive being 0–1% MAF and the most inclusive being 0–5%. For each MAF and variant set, we assessed whether any genes deviated from expectation as demonstrated by the diagonal line. The only gene that showed enrichment was BTNL2 ( P =7.0 × 10 −8 , Fisher’s exact test). Full size image Classical HLA allele imputation We imputed four-digit classical HLA alleles and amino acid sequences in 162 CIAG cases and 4,319 controls of European ancestry from a reference panel of 5,225 individuals using SNP2HLA [15] . The cases, mainly of northwestern European and Ashkenazi Jewish ancestry, were well-matched to controls ( Supplementary Fig. 5 ). Two independent loci are associated with CIAG after multiple-testing correction ( Fig. 4 ). The top signal is an amino acid change in HLA-DQB1 (126Q) that is in strong LD with HLA-DQB1*05:02 ( P =4.7 × 10 −14 , OR=0.19, 95% CI=0.12–0.29). After conditioning on HLA-DQB1 126Q, a genome-wide significant signal in HLA-B remains (alanine to threonine at residue 158, P cond =1.54 × 10 −8 , OR=3.11, 95% CI=2.1–4.6). No other statistically significant loci remain after conditioning on both HLA-DQB1 126Q and HLA-B 158T ( Supplementary Data 3 ). 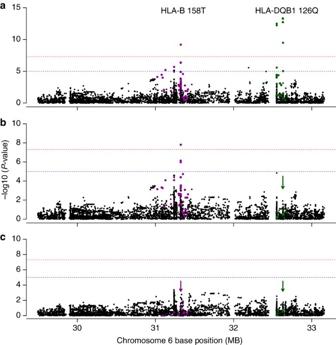Figure 4: Manhattan plot of the MHC region from HLA imputation. This figure shows the association results of CIAG to imputed HLA classical alleles, amino acids and SNPs for 161 cases and 4,300 controls. (a) The top signal is from a single amino acid inHLA-DQB1(126Q) (P=4.7 × 10−14, OR=0.19, logistic regression). All variants with anR2>0.1 withHLA-DQB1126Q are coloured green. (b) After conditioning onHLA-DQB1126Q as demonstrated by the green arrow, the top signal is a single amino acid inHLA-B(158T) (Pcond=1.54 × 10−8, OR=3.11, logistic regression). All variants with anR2>0.1 withHLA-B158T are coloured purple. (c) After conditioning onHLA-DQB1126 Q andHLA-B158T (purple and green arrows), no genome-wide significant loci remain. Figure 4: Manhattan plot of the MHC region from HLA imputation. This figure shows the association results of CIAG to imputed HLA classical alleles, amino acids and SNPs for 161 cases and 4,300 controls. ( a ) The top signal is from a single amino acid in HLA-DQB1 (126Q) ( P =4.7 × 10 −14 , OR=0.19, logistic regression). All variants with an R 2 >0.1 with HLA-DQB1 126Q are coloured green. ( b ) After conditioning on HLA-DQB1 126Q as demonstrated by the green arrow, the top signal is a single amino acid in HLA-B (158T) ( P cond =1.54 × 10 −8 , OR=3.11, logistic regression). All variants with an R 2 >0.1 with HLA-B 158T are coloured purple. ( c ) After conditioning on HLA-DQB1 126 Q and HLA-B 158T (purple and green arrows), no genome-wide significant loci remain. Full size image HLA-DQB1 and HLA-B explains the MHC signal better than BTNL2 To determine whether the BTNL2 signal is independent of the HLA-B 158T and HLA-DQB1 126Q signals, we analysed samples with imputed HLA alleles and genotyped BTNL2 variants (146 CIAG cases and 3,364 controls). In conditional analyses, we observed that the most-associated BTNL2 variant (rs28362679) was in high LD with HLA-DQB1 126Q ( R 2 =0.618) and the other BTNL2 variant (rs143211074) had a low correlation with HLA-B 158T ( R 2 =0.042) ( Supplementary Fig. 6 ). To determine whether the association in the region was better explained by the two variants in BTNL2 or the two HLA alleles, we compared the likelihoods of models with HLA-DQB1 126Q and HLA-B 158T predicting CIAG compared with a model with the two BTNL2 variants. The combination of HLA-DQB1 126Q and HLA-B 158T is 27,000 times more likely to explain the MHC association with CIAG than the two BTNL2 variants. We also looked at whether a model including one or both BTNL2 variants in addition to HLA-DQB1 126Q and HLA-B 158T explained the association better than HLA-B and HLA-DQB1 alone. We found including rs143211074 in the model was 13 times more likely to explain the association than the two-component model of HLA-B and HLA-DQB1 , but there was no improvement when we added rs28362679. These results indicate that rs143211074 could be independently associated with CIAG, but the more likely explanation is that rs143211074 is tagging an HLA haplotype that is not genome-wide significant on its own (given that rs143211074 and HLA-DRB1*04:02 are highly correlated with R 2 =0.77). HLA sequence alignment We used the IMGT/HLA database [16] ( http://www.ebi.ac.uk/ipd/imgt/hla ) to determine which classical alleles correspond to HLA-DQB1 126Q and HLA-B 158T and to align these results with previous candidate gene studies of CIAG. Since having a glutamine at position 126 in HLA-DQB1 is protective for CIAG, the most common high-risk allele is HLA-DQB1*05:02 which has a histidine at position 126. This is consistent with prior reports of an association of CIAG with HLA-DQB1 6672G>C (a variant in strong LD with HLA-DQB1*05:02 ) [4] , [5] . HLA-B*38 , HLA-B*39 and HLA-B*67 are the most common alleles with a threonine at position 158 in the protein sequence (consistent with previous reports although none met contemporary significance levels) [3] , [4] , [8] . Our results cannot differentiate whether the amino acids we identified are causal or whether the overall configuration of these genetically related isoforms confers risk for CIAG. CIAG severity by HLA-B and HLA-DQB1 carrier status Finally, we tested for differences in CIAG severity (as indexed by minimum absolute neutrophil count, ANC) according to risk allele status of HLA-DQB1 and HLA-B among 149 cases with these data. Cases who were carriers of HLA-B 158T demonstrated significantly lower ANC than noncarriers ( P <0.01, Fig. 5 ). However, as nearly all cases with substantial Ashkenazi Jewish ancestry carried the HLA-B 158T allele ( Supplementary Fig. 7 ), it is not possible to determine conclusively whether some of this signal could be driven by an unexplored feature of ascertainment or population difference. Hence we repeated the analysis after excluding cases with Ashkenazi Jewish ancestry (PC1>0.02) and subsequently correcting the phenotype for ancestry and sample cohort and observed a consistent effect but of reduced significance ( P =0.049) owing to reduced power because of the number of 158T alleles excluded ( Supplementary Fig. 8 ). Similar analyses of time to onset of CIAG were not significant (data not shown). 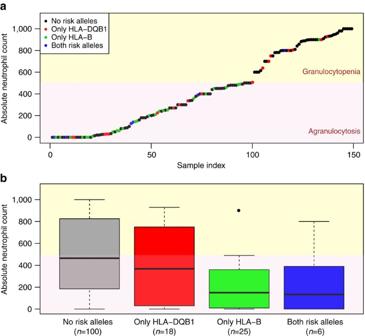Figure 5: Absolute neutrophil count stratified by HLA risk allele carrier status. (a) For cases in which the lowest recorded absolute neutrophil count (ANC) data were available, we ordered samples by the ANC and coloured the points by their imputed carrier status ofHLA-DQB1126Q andHLA-B158T (black=no risk alleles, red=only a carrier ofHLA-DQB1risk alleles as tagged by 126Q, green=only a carrier ofHLA-B158T, blue=carrier of bothHLA-DQB1andHLA-Brisk alleles). The background colours demonstrate the clinical definitions for agranulocytosis (red: ANC<500) and severe granulocytopenia (yellow: 500≤ANC≤1000). (b) The same data are shown as a box plot to demonstrate thatHLA-B158T carriers demonstrate a trend towards lower ANC than noncarriers ofHLA-B158T. Figure 5: Absolute neutrophil count stratified by HLA risk allele carrier status. ( a ) For cases in which the lowest recorded absolute neutrophil count (ANC) data were available, we ordered samples by the ANC and coloured the points by their imputed carrier status of HLA-DQB1 126Q and HLA-B 158T (black=no risk alleles, red=only a carrier of HLA-DQB1 risk alleles as tagged by 126Q, green=only a carrier of HLA-B 158T, blue=carrier of both HLA-DQB1 and HLA-B risk alleles). The background colours demonstrate the clinical definitions for agranulocytosis (red: ANC<500) and severe granulocytopenia (yellow: 500≤ANC≤1000). ( b ) The same data are shown as a box plot to demonstrate that HLA-B 158T carriers demonstrate a trend towards lower ANC than noncarriers of HLA-B 158T. Full size image Modelling of clozapine binding to HLA-B The associations of HLA-DQB1 and HLA-B with CIAG are biologically plausible. HLA-DQB1 is part of the MHC Class II antigen-presentation pathway and has been associated with autoimmune diseases (for example, rheumatoid arthritis) [17] and a range of immunogenetic phenomena (for example, allergic sensitization, human papillomavirus seropositivity and chronic hepatitis B infection) [18] , [19] , [20] . HLA-B is an important component of the MHC Class I antigen-presentation pathway and a ‘hot spot’ for serious adverse drug reactions including flucloxacillin-induced liver injury [21] , carbamazepine-induced Stevens–Johnson syndrome [22] , and abacavir hypersensitivity syndrome [23] . For several of these adverse drug reactions, the mechanism appears to be off-target binding of a drug molecule to the antigen-binding cleft of the HLA-B protein [23] . Similar to what has been done for abacavir [23] , we used a molecular docking approach to determine that clozapine binds with relatively high affinity to the putative HLA-B*39 antigen-presenting peptide groove when there is a threonine at position 158 ( Fig. 6 ). Docking simulations also suggested a potential for clozapine to bind in the pockets of HLA-B*57:01 and HLA-B*35:08 with predicted affinities much higher than that for multiple other HLA-B variants ( Supplementary Fig. 9 ). As a negative control, docking studies showed that clozapine had low binding affinities for the antigen-presenting pockets of HLA-A proteins. 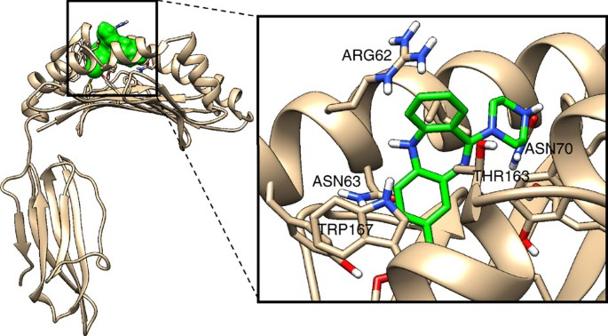Figure 6: Predicted binding pose of clozapine in the antigen-presenting pocket ofHLA-B*39. Docking of clozapine into the putative antigen-binding pocket of the homology model ofHLA-B39identified a binding pose (shown in this figure) with the highest predicted binding affinity. Residues in the protein-binding pocket involved in specific interactions with clozapine are annotated. Figure 6: Predicted binding pose of clozapine in the antigen-presenting pocket of HLA-B *39. Docking of clozapine into the putative antigen-binding pocket of the homology model of HLA-B39 identified a binding pose (shown in this figure) with the highest predicted binding affinity. Residues in the protein-binding pocket involved in specific interactions with clozapine are annotated. Full size image In conclusion, we identified two independent loci in the MHC region that are associated with CIAG: HLA-DQB1 and HLA-B . These findings are consistent with previous results but the evidence is now much stronger in this comprehensive analysis. Moreover, we localized the signal to two amino acids ( HLA-DQB1 126Q and HLA-B 158T), but cannot distinguish whether these amino acids are causal or if the overall configuration of the alleles confers risk for CIAG. Although these data greatly clarify the contributions of HLA variation to CIAG, the ORs do not immediately suggest clinical application in screening. If we consider a genetic test that was positive if an individual carried either risk factor, the sensitivity and specificity of such a test would be 0.36 and 0.89. Because more than half of the cases do not carry these two relatively infrequent risk factors, a predictive test based solely on HLA-DQB1 and HLA-B could not define a truly ‘safe’ group for clozapine use. We note that seven CIAG cases (4.3%) carried two risk alleles, suggesting that this combination had particularly high risk compared with the population expectation of 0.3–0.4%. These genetic insights could further help in understanding the biological processes underlying CIAG and, as other non-genetic and genetic risk factors for CIAG are identified, constitute an important component of tests to screen patients for the safer use of clozapine. Ethical statement The study was approved by Institutional Review Boards at the University of North Carolina ( http://research.unc.edu/offices/human-research-ethics ) and at Massachusetts General Hospital ( http://healthcare.partners.org/phsirb ). Research was carried out in accordance with the Declaration of Helsinki. Written informed consent was obtained from all the participants (or legal guardians, if applicable). Sample description We formed the Clozapine-Induced Agranulocytosis Consortium (CIAC) to further this effort by bringing together nearly all investigators in the area and to ascertain new cases. CIAG (clozapine-induced agranulocytosis/granulocytopenia) cases developed agranulocytosis (ANC<500 mm −3 ) or granulocytopenia (500≤ANC≤1,000 mm −3 ) while taking clozapine and without a known medical condition that increases risk for agranulocytosis (for example, haematological disorder or autoimmune disease). There were 98 cases with agranulocytosis (60.1%), 61 cases with granulocytopenia (37.4%) and four cases (2.5%) included on the basis of clinical judgment due to a precipitous drop in ANC to <1,500 mm −3 while being intensively monitored. We allowed any primary psychiatric diagnosis (although most subjects had schizophrenia or schizoaffective disorder) and any reported ancestry was allowed. Heterogeneity due to ANC threshold, diagnosis and ancestry was addressed analytically. Subjects were identified in two ways. Opportunistic ascertainment was via a broad survey of colleagues to identify all worldwide samples in existing CIAG collections that allowed rapid and efficient identification of existing CIAG cases and controls exposed to clozapine without CIAG. This included cases from the International Severe Adverse Events Consortium (iSAEC, http://www.saeconsortium.org ). Systematic assessment included identification of additional cases from the Novartis and Teva clozapine registries ( https://www.clozarilcare.com/care , https://www.clozapineregistry.com ), and the electronic pharmaceutical record from the Pennsylvania state hospital system. Briefly, we contacted the physician of record to confirm an episode of CIAG, the physician then obtained permission from the potential subject to release contact information, and we then contacted the subject to attempt recruitment into this study. We attempted to obtain and review medical records for all subjects. Using a standardized review form, we abstracted demographic data, clinical diagnosis, and clozapine dosage, exposure duration and the lowest ANC. Two senior CIAC clinicians evaluated all available data to verify CIAG case status. Most DNA samples were extracted from peripheral venous blood; a subset of DNA samples were from lymphoblastoid cell lines or oral sources. Most samples were subjected to standard quality control procedures (DNA quantification, electrophoresis to assess degradation and genotyping a ‘fingerprint’ of 25 common SNPs using a Sequenom iPLEX panel). Genotype data confirmed that all subjects were independent and of European ancestry (see below). A combination of clozapine-treated and untreated controls was used to increase statistical power. Clozapine-treated controls had received clozapine for over 1 year with no documented ANC<1,500 mm −3 and no medical condition with an increased risk of agranulocytosis. Ascertainment of clozapine-treated controls was performed in the same manner as for the cases. Untreated controls were broadly consented population controls ascertained in unrelated disease and cohort studies. Allele frequency data from the NHLBI Exome Sequencing Project (ESP) were also used. Generation of genome-wide array data A total of 385 samples from CIAC (135 cases and 249 treated controls) were genotyped on the Illumina OmniExpress array at Duke University. We supplemented the CIAC data with 839 untreated population controls from the United Kingdom Blood Service cohort who were genotyped on the Illumina OmniExpress platform at the Broad Institute. In addition, 26 case samples from the International Serious Adverse Events Consortium (iSAEC, http://www.saeconsortium.org ) were genotyped at Duke University on the Illumina Human610-Quadv1_B platform. These data were merged with 108 untreated population controls from the NIMH repository genotyped on the Illumina 550K array at the University of Michigan. Genotype calls were generated using the GenomeStudio software from Illumina. All samples had a call rate >98% and an inbreeding coefficient between −0.2 and 0.2. SNPs were included if the call rate was >98%, were in Hardy–Weinberg equilibrium ( P control >1 × 10 −6 , P case >1 × 10 −10 ) and the call rate difference between cases and controls was <0.02. Samples were unrelated and of European ancestry via multidimensional scaling [24] . We used SHAPEIT [25] , [26] and IMPUTE2 (ref. 27 ) to impute genotypes for all SNPs using 1000 Genomes Project data as a reference panel. The imputation reference set was 2,186 phased haplotypes from the 1000 Genomes Project (August 2012, 30,069,288 variants, release ‘v3.macGT1’, http://mathgen.stats.ox.ac.uk/impute/data_download_1000G_phase1_integrated.html ). Imputation was done for each platform separately (OmniExpress, I550K/I610K) to avoid platform-based batch effects in imputation. Generation of whole-exome sequencing data We sequenced 41 CIAC cases and 26 iSAEC cases at Duke University. Exome sequence from CIAC cases was captured using Agilent SureSelect 50 MB kits (Santa Clara, CA) and sequenced using Illumina HiSeq 2000 (San Diego, CA) for paired-end 100 bp reads. The iSAEC samples were sequenced several years earlier using Agilent SureSelect kits (Santa Clara, CA) and Illumina GAII for paired-end reads (San Diego, CA). For controls, we used data from 376 phenotypically normal controls who had been exome sequenced at the Broad Institute [28] . All raw FASTQ data were processed using the same Picard pipeline [29] , [30] and genotype calls were generated for all data jointly using the GATK Unified Genotyper tool [31] to avoid batch effects. Individual genotype calls were filtered by requiring read depth ≥10, genotype quality score ≥30 and meeting-specified allelic balance criteria (based on genotype: for 0/0, 0–0.3; for 0/1, 0.3–0.7; and for 1/1, 0.7–1.0). All variants were required to have a GATK PASS rating, to be biallelic, not to have a significant difference in call rate between cohorts ( P >0.01, eliminates biases due to a variant being sequenced in one cohort but not in the other), and not to be an insertion/deletion variant. Samples were required to have a call rate >95%, <600 singleton calls and a Ti:Tv ratio between 3.1 and 3.4. The first 10 principal components (PCs) were computed using PLINK with 14,466 independent variants with an MAF >5% and not located in the MHC region. Generation of exome array data We genotyped deleterious exonic variation and a comprehensive set of MHC tag SNPs using the Illumina HumanExome array (v1.0, http://genome.sph.umich.edu/wiki/Exome_Chip_Design ). Initial genotyping was conducted at Duke University and genotype calls were made using GenomeStudio (v2010.3, genotyping module v1.8.4) using the default Illumina cluster file. Samples were removed for missingness >1% (based on common SNPs with MAF >5%) or genome-wide heterozygosity outside the range of 0.1–1.2% (based on rarer SNPs with MAF <5%) using the original GenomeStudio calls. Cases that failed quality control ( N =23) were re-genotyped at the Broad Institute on the Illumina HumanExome array (v1.1); genotype calling and quality control were the same as for the Duke data except that a custom cluster file and a missingness threshold >2% were used. We then used zCall to recover rare genotypes [32] . After removing poorly performing samples, individual SNPs from the Duke data were included if they had a call rate >97% from the original GenomeStudio calls, a HWE P -value >1 × 10 −5 and a call rate >99.5% calculated from the zCalls. For the Broad data, more lenient call rate thresholds were used due to the small number of samples (GenomeStudio calls >75%, zCalls >95%). The passing exome array data were merged with population controls of European ancestry broadly consented for biomedical studies. These controls included samples from the NIMH repository ( n =1,037) [33] , POPRES ( n =703) [21] , the Prospective Registry in IBD Study ( n =254) [34] , the 1000 Genomes Project ( n =449) [35] and controls ascertained for an age-related macular degeneration study ( n =704) [36] . Quality control for the shared controls was similar to the steps for the CIAC data, except that a call rate of 99% was used [36] . The final data set included only SNPs passing quality control in all cohorts. We removed one member of putative relative pairs ( >0.2) and used EIGENSOFT [37] to calculate the first 10 PCs based on 16,621 SNPs (MAF >5%, excluding the extended MHC region (chr6:25–35 mb), and following LD pruning). Two hundred and thirteen out of 3,366 controls were ascertained for not having CIAG. HLA allele imputation HLA classical alleles and amino acids were imputed using BEAGLE [38] for exome array data or IMPUTE2 (ref. 27 ) for genome array data with a reference set of 5,225 samples from the Type 1 Diabetes Genetics Consortium [15] . The imputation accuracy using this reference panel is extremely high. For example, the SNP2HLA authors found that the accuracy of HLA-B*38:01 was 99.8%, HLA-B*39:01 was 99.8% and HLA-B*39:06 was 99.9% using the same set of MHC tag SNPs present on the Illumina HumanExome array compared with direct genotyping of these variants [15] . We also confirmed the accuracy of imputation of HLA-DQB1*05:02 by SNP2HLA using existing data for 19 samples that had PCR-based sequencing of HLA-DQB1 6672G>C, which is in strong LD with HLA-DQB1*05:02 (ref. 7 ): Thirty-seven out of 38 imputed HLA-DQB1*05:02 calls were concordant with the PCR-based sequencing results. Genome-wide common variant association study PCs were calculated using EigenSoft with the merged OmniExpress and I550K/I610K imputed data sets. SNPs used to calculate the PCs were independent (LD pruned) and did not include the MHC (chr6:25–35 Mb). We tested the first 20 PCs for phenotype association (using logistic regression) and evaluated their impact on the genome-wide test statistics using λ , a measure of how much the observed distribution of P values deviates from the expected distribution of P values. Five PCs (1–4 and 12) were included in all association analyses. The first four PCs were selected because it is a standard practice to include the first four PCs in analyses to account for ancestry and, of PC5–PC20, PC12 was the only PC associated with case–control status ( P <0.05). We performed a mega-analysis between the OmniExpress data and the I550K/I610K imputed dosage data using PLINK with PCs (described above) as covariates for logistic regression. SNPs with an INFO score ≥0.6 (metric of imputation quality for a SNP) and MAF ≥1% in controls were considered passing. We did not observe any batch effects due to multiple platforms or confounding due to population ancestry as indicated by a value of λ =1.047 and no false positive results ( Supplementary Fig. 1 ). Immune-mediated SNP Enrichment To determine whether our GWAS results show any indication of signal in loci known to be associated with autoimmune diseases, we randomly drew P values from the GWAS results above to create an expected null distribution. To make this comparison more representative in terms of power per SNP, random draws were only taken from the subset of variants with MAF >0.05 and INFO >0.8 (6,752,294 SNPs). We drew 100 sets of 838 SNPs and compared the distribution of P values to those observed in a curated list of 838 associations to immune-mediated and autoimmune disease curated from the NHGRI GWAS catalogue. The comparison demonstrated that CIAG association to known immune-mediated SNPs was not distinguishable from random draws of SNPs. Exome-wide rare variant association study Because we had data from different platforms for rare exonic variants (exome sequencing, array and allele counts from the ESP [11] , available at http://evs.gs.washington.edu/EVS ), we used the following procedure to combine allele counts. If a variant was assayed on multiple platforms, we ensured that the MAFs between the controls did not differ ( P >0.001). If the MAFs in controls were not compatible, we removed data in the following order: ESP, exome array and exome sequencing. For each variant, we added allele counts for each technology in both cases and controls and used Fisher’s exact test on the combined sample to test for significance. Variants were functionally annotated using the Variant Effect Predictor tool from Ensembl [39] . We then divided the annotations into three categories. The most restrictive grouping included all nonsense and splice-region variants. The intermediate grouping included all nonsense, splice-region and missense variants annotated as probably damaging by PolyPhen-2 (ref. 40 ). The least restrictive grouping included all nonsense, splice-region, missense and untranslated region variants. To test for an excess burden of rare and functional variants, we used Fisher’s exact test where the variable of interest is the number of carriers of a functional variant. We used the number of carriers of a functional variant instead of the total minor allele count as the testing variable to account for LD between variants. MHC association analysis We used imputed HLA classical alleles from all the samples that were genotyped on the exome array. For the remaining samples that were not genotyped on the exome array, we imputed HLA classical alleles from either OmniExpress or I500K. PCs were calculated from 6,000 independent markers that were present on all three platforms to obtain one consistent set of PCs for all samples using PLINK ( Supplementary Fig. 5 ). We merged the imputed dosage data from all the three platforms to do a mega-analysis and used logistic regression to calculate association test statistics for each imputed allele using the first 10 PCs as covariates in PLINK to account for any confounding due to population structure. For conditional analyses, we used the dosage of the conditioning marker as an additional covariate in the analysis. Model comparison We used R to compute the log-likelihood of a logistic regression model consisting of either the top two BTNL2 missense variants or HLA-DQB1 126Q and HLA-B 158T dosages with the first 10 PCs as covariates in 144 cases and 3,355 controls. We also explored whether adding one or both BTNL2 variants improved the model consisting of HLA-DQB1 126Q and HLA-B 158T. LD calculations We used PLINK to calculate the R 2 between each pair of variants in both cases and controls who had BTNL2 and HLA imputation data ( n =146 cases and 3,364 controls). Haploview [41] was used to plot the LD between the top BTNL2 variants, HLA-B 158T, HLA-DQB1 126Q alleles and the top HLA-DRB1 alleles ( *04:02 and *16:01 ). Wilcoxon rank-sum tests We used a Wilcoxon Rank-Sum test in R to determine whether the ANC distribution between carriers and noncarriers of HLA risk alleles was different in cases who had a lowest recorded ANC ≤1,000 ( n =149). To correct for covariates, we used the residuals of the regression between ANC and the PCs and cohort indicator as the quantitative variable for the Wilcoxon rank-sum test ( Supplementary Fig. 8 ). For samples with dosage, treatment duration and minimum ANC available ( n =92), we calculated the correlation between these variables. ANC is moderately correlated with treatment duration ( R 2 =0.165) and weakly correlated with clozapine dosage ( R 2 =0.035). Treatment duration is moderately correlated with dosage ( R 2 =0.229). Carrier status was determined using the best guess genotype for the HLA-B 158T and HLA-DQB1 126Q alleles. Copy number variation analysis To generate CNV genotypes, we applied PennCNV to the Illumina OmniExpress data. We removed any samples that had a log R ratio standard deviation >0.3 or that were above the 95th percentile for the number of CNV calls leaving 134 cases and 242 controls. CNVs included for analysis were required to have >10 SNP probes, >20 kb in length, <50% overlap with large genome gaps and with MAF <1% in controls. We used PLINK to test for CIAG association using the ‘--cnv-test-2sided’ command with significance determined using 100,000 permutations. The family-wise corrected P values were examined. No rare CNV was significantly associated with CIAG (data not shown). Molecular docking We used the Maestro 2012 software suite (Schrödinger, http://www.schrodinger.com ) to build a homology model of HLA-B39 using the protein structures of HLA-B*08 (Protein Data Bank, PDB, http://www.wwpdb.org , code=3SPV, resolution 1.30Å) and HLA-B*41 (PDB code=3LN4, resolution 1.30 Å) as templates. We also used a multiple sequence alignment encompassing HLA-B*08 , B41 and B38 . Clozapine was docked into the antigen-presenting site of the predicted structure of HLA-B39 using the Glide program in extra-precision docking mode (Glide XP). Ionizable groups were first converted to their most probable charged forms at pH 7.4 using the LIGPREP software within Maestro. The binding region was defined by a 10 × 10 × 10 Å box centred on the B39 pocket. A scaling factor of 0.8 was applied to the van der Waals radii. Default settings were used for all the remaining parameters. The docking poses were energy-minimized with Macromodel in the OPLS2005 force field with flexible ligand and rigid receptor. The refined poses were re-ranked on the basis of the calculated interaction energy. The lowest-energy pose was selected and rescored in the active site using GlideScore XP. Clozapine was also docked in the antigen-presenting sites of HLA-B*57:01 (PDB code=3VRI), HLA-B*35:08 (PDB code=3BWA) and the binding pockets of other HLA-A and HLA-B proteins. How to cite this article: Goldstein, J. I. et al . Clozapine-induced agranulocytosis is associated with rare HLA-DQB1 and HLA-B alleles. Nat. Commun. 5:4757 doi: 10.1038/ncomms5757 (2014).